Visualization of poly(ADP-ribose) bound to PARG reveals inherent balance betweenexo- andendo-glycohydrolase activities Poly-ADP-ribosylation is a post-translational modification that regulates processes involved in genome stability. Breakdown of the poly(ADP-ribose) (PAR) polymer is catalysed by poly(ADP-ribose) glycohydrolase (PARG), whose endo -glycohydrolase activity generates PAR fragments. Here we present the crystal structure of PARG incorporating the PAR substrate. The two terminal ADP-ribose units of the polymeric substrate are bound in exo -mode. Biochemical and modelling studies reveal that PARG acts predominantly as an exo -glycohydrolase. This preference is linked to Phe902 (human numbering), which is responsible for low-affinity binding of the substrate in endo -mode. Our data reveal the mechanism of poly-ADP-ribosylation reversal, with ADP-ribose as the dominant product, and suggest that the release of apoptotic PAR fragments occurs at unusual PAR/PARG ratios. Poly-ADP-ribosylation is a reversible post-translational modification that regulates a variety of cellular functions involved in genome stability [1] , [2] , [3] , [4] . Poly(ADP-ribose) (PAR) synthesis is achieved by poly(ADP-ribose) polymerases (PARPs), which, by using NAD as substrate, link repeating ADP-ribose units via unique O-glycosidic ribose–ribose bonds [5] . Efficient and timely breakdown of the PAR polymer is catalysed by a PAR glycohydrolase (PARG), and PARG depletion results in embryonic lethality in mouse models, as well as increased radiosensitivity and chemosensitivity in cells, making PARG an attractive therapeutic target [6] , [7] , [8] . The complex chemical nature of the poly(ADP-ribose) polymer has limited the understanding of the structure and recognition of this signalling molecule. Recent structure determination of PARG from bacterial, protozoan and mammalian sources [9] , [10] , [11] , [12] revealed that these enzymes essentially consist of a macrodomain ADP-ribose-binding module [13] , elaborated upon through insertion of the highly conserved and PARG-specific catalytic loop (containing the key catalytic residues), and both N- and C-terminal extensions. Canonical eukaryotic PARGs are more complex when compared with their prokaryotic counterparts. In terms of size, canonical PARGs are bigger and contain a significantly larger accessory domain to the aforementioned, essential substrate-binding macrodomain ( Supplementary Fig. S1 ). Furthermore, the bacterial type PARGs have recently been shown to act solely in an exo-glycohydrolase mode [9] , whereas canonical PARGs have been reported to exhibit both endo- and exo-glycohydrolase activities [14] . PARG is unable to cleave the ester bond linking the proximal ADP-ribose unit directly to proteins [9] . Although the enzymatic activity that catalyses this step of PAR catabolism has been detected in mammalian cell extracts 30 years ago, the proteins responsible remained unknown until very recently [15] , [16] , [17] , [18] . The deficiency in the proteins demodifying mono(ADP-ribosyl)ated PARP substrates in cells leads to a severe neurodegeneration disease in humans [16] , [19] . To provide detailed understanding of the inherent endo- and exo-glycohydrolase activities of canonical PARGs, we set out to determine the structure of an inactive PARG in complex with the PAR substrate. Crystal structure determination of the E256Q Tetrahymena thermophila PARG in complex with PAR fragments surprisingly yielded only exo-glycohydrolase-mode complexes. The inherent preference for exo- (as opposed to endo-) binding is linked to the presence of the conserved residue Phe902 (human numbering), and this is confirmed by detailed studies of product profiles for canonical PARGs. We conclude that, in contrast to bacterial PARG, canonical PARGs can act as endo-glycohydrolases. The balance between exo- and endo-activity is likely to be a function of the PARG/PAR ratio, offering the possibility that apoptotic PAR fragments are only formed at unusual PARG/PAR ratios. Crystal structure of the inactive TTPARG with PAR To understand poly-ADP-ribose binding by canonical PARGs, we prepared homogenous PAR fragments. PAR was prepared by enzymatic synthesis using the activity of PARP Tankyrase1 as described [20] , which assures the production of biologically relevant polymers. The PAR fragments were resolved by anionic chromatography at single-nucleotide resolution, providing sufficient amounts of homogenous PAR fragments of defined lengths for the envisioned structural studies ( Supplementary Fig. S2 ). Size identity of PAR fragments was confirmed by mass spectrometry. The inactive E256Q TTPARG mutant was co-crystallized with a series of defined length PAR oligomers, ranging from a 6-mer to a 16-mer fragment. Crystals were obtained in a range of conditions, for each of the PAR polymers tested. In all cases, the same crystal packing was observed, regardless of PAR polymer size or mother liquor composition. No significant difference in the corresponding structures was observed, and we report the highest resolution structure obtained to 1.46 Å for a E256Q TTPARG in complex with a PAR 9 (PDB code 4L2H). Compared with previously determined TTPARG structures [10] , changes in the TTPARG protein structure are minor and are probably due to the distinct crystal packing obtained for the PARG–PAR 9 complex. The bound poly-ADP-ribose can clearly be discerned from the electron density, but only the two terminal ADP-ribose units are visible ( Fig. 1a ). The terminal ADP-ribose moiety occupies a position similar to that observed for the product ADP-ribose molecule. The ribose–ribose O-glycosidic linkage between both ADP-riboses is clearly visible and is positioned in close proximity of the Gln256 side chain ( Fig. 1b ). In contrast to the interactions between Asn250 and Glu255 and the terminal ribose’, no direct interactions are observed between protein and the n-1 ribose’. The 3-OH group of the latter is within hydrogen bonding distance of the terminal n ribose’ 3-OH (in turn bound by Asn240) and a water molecule (referred to as W2). The W2 is bound by the Gly246 amide nitrogen and the n ribose’ 2-OH group (bound to Glu255). The n-1 adenosine is sandwiched between Val253 and water molecules that interact with Arg164. Direct hydrogen bonding interactions between the Leu252 amide nitrogen and the n-1 adenosine N11, as well as the Ser297 side chain and the n-1 adenosine N10, can also be observed. A few polar interactions occur between the protein and the n-1 diphosphate, including the amide nitrogen backbone, and side chain of Asn250. As a consequence, starting with the n-1 α-phosphate towards the N-2 ADP-ribose group of the PAR chain, electron density rapidly becomes weaker, signifying high levels of flexibility in the bound PAR from the n-1 α-phosphate onwards. Beyond the n-1 β-phosphate, electron density is reduced to background level, corresponding to the large crystal solvent channel that lines the TTPARG active-site region ( Supplementary Fig. S3 ). The latter region is sufficiently large to contain the remaining disordered PAR section. 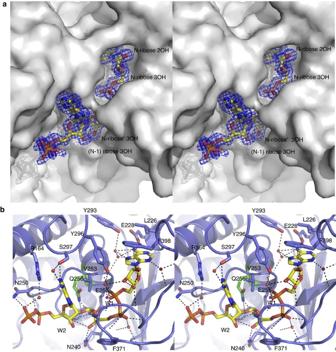Figure 1: Crystal structure of a PARG–PAR complex. (a) Stereoview of the solvent-accessible surface of PARG in grey with the bound PAR at the active-site surface shown in atom-coloured sticks. The 2FoFcelectron density corresponding to the ordered region of PAR is shown in a blue mesh (contour level 1 sigma). (b) Stereoview of the PARG active site. Residues involved in direct contacts with the PAR ligand are shown in atom-coloured sticks. The mutated Glu256 is shown with green rather than with light blue carbons. Hydrogen bonds between ligand and protein or structural waters are indicated by dotted lines. Figure 1: Crystal structure of a PARG–PAR complex. ( a ) Stereoview of the solvent-accessible surface of PARG in grey with the bound PAR at the active-site surface shown in atom-coloured sticks. The 2F o F c electron density corresponding to the ordered region of PAR is shown in a blue mesh (contour level 1 sigma). ( b ) Stereoview of the PARG active site. Residues involved in direct contacts with the PAR ligand are shown in atom-coloured sticks. The mutated Glu256 is shown with green rather than with light blue carbons. Hydrogen bonds between ligand and protein or structural waters are indicated by dotted lines. Full size image Comparison of the TTPARG–PAR 9 structure with the recently published human PARG structure [12] reveals that the majority of PARG–PAR interactions are conserved across eukaryotic PARGs ( Supplementary Fig. S4 ). The few differences that are observed are located in the vicinity of the n-1 ADP-ribose unit, providing further evidence that this region does not significantly contribute to PAR binding ( Fig. 2 ). Indeed, mutations of residues implicated in the binding of the n-1 ADP-ribose suggested by the TTPARG–PAR crystal structure, or, by analogy, a human PARG–PAR model, have little to no effect on PARG catalytic activity ( Fig. 2 ). In contrast, mutations of residues implicated in the binding of the n adenosine moiety in humans and TTPARGs significantly diminish activity, suggesting that analogous PAR binding mode also occurs in human PARG. 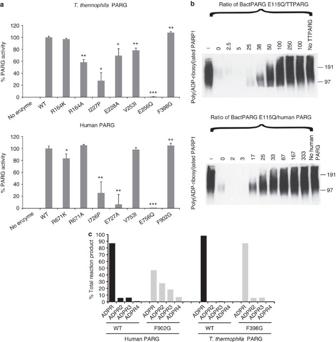Figure 2: PARG mutagenesis and PAR termini protection by bactPARG confirms the PARG–PAR model. (a) Activity of theT. thermophilaPARG WT and mutants and the corresponding human PARG mutants. Error bars represent s.d. (n=3) (*P<0.05; **P<0.01; ***P<0.001) obtained using pairedt-test. (b) Inhibition of glycohydrolase activity for both human andT. thermophilaPARGs using PARP1-generated PAR substrate with bactPARG Glu115Gln. (c) Distribution of exo- and endo-glycohydrolase products obtained after treatment with wt and mutant human andT. termophilaPARGs, as determined by LC/MS (see alsoSupplementary Fig. S6). Figure 2: PARG mutagenesis and PAR termini protection by bactPARG confirms the PARG–PAR model. ( a ) Activity of the T. thermophila PARG WT and mutants and the corresponding human PARG mutants. Error bars represent s.d. ( n =3) (* P <0.05; ** P <0.01; *** P <0.001) obtained using paired t -test. ( b ) Inhibition of glycohydrolase activity for both human and T. thermophila PARGs using PARP1-generated PAR substrate with bactPARG Glu115Gln. ( c ) Distribution of exo- and endo-glycohydrolase products obtained after treatment with wt and mutant human and T. termophila PARGs, as determined by LC/MS (see also Supplementary Fig. S6 ). Full size image PARG binds PAR in an exo -glycohydrolase binding mode The observed binding mode corresponds to a PARG exo-glycohydrolase activity, and, given the fact that previous studies suggested potential PAR conformations corresponding to endo-glycohydrolase activity were compatible with canonical PARG structures [10] , [11] , [12] , comes as a surprise. The 2-OH group of the terminal ribose’ is indeed solvent exposed ( Fig. 1a ), suggesting that a further n+1 unit could fit at the PARG surface. The crystal packing is also such that a large solvent channel runs along the PARG active-site surface, and is thus unlikely to influence the observed PAR conformation ( Supplementary Fig. S3 ). We re-evaluated the modelling of a PAR trimer using the new TTPARG–PAR structure and compared the average architectures of an exo-glycohydrolase and an endo-glycohydrolase binding mode during molecular dynamics (MD) simulations ( Fig. 3a ). These reveal that although binding of an additional n+1 unit is indeed possible, this requires a reorientation of the n ribose’ to allow for the presence of the additional n+1 ribose’ unit and avoid steric clashes with conserved Phe398 ( Fig. 3b ). This in turn leads to a reorientation of the n adenosine, which is no longer able to maintain a series of polar interactions with the side chain of Glu228 and the amide nitrogen of Ile227. In addition, a water-mediated interaction with Lys365 and Cys396 backbone atoms is also disrupted. The disruption of complementarity between the PARG active site and the n adenosine provides a likely explanation for the observed preference to bind the PAR terminus ( Table 1 ). Given the fact that only an exo-glycohydrolase conformation was observed for different PAR lengths, with the longest oligomer reaching 15 ADP-ribose units (which contains only 1 terminal residue, compared with 13 intermediate positions), this preference can be estimated to be at least 100-fold. 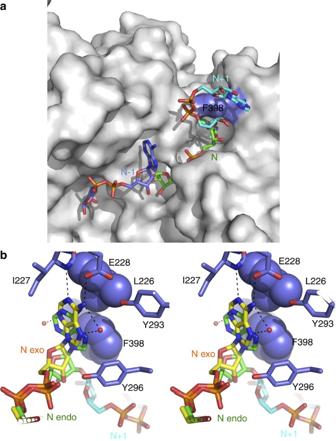Figure 3: Model of the PARG–PAR complex in endo-glycohydrolase mode. (a) Solvent-accessible surface of PARG in grey (the position of Phe398 is shown in blue) with a PAR3modelled in an endo-glycohydrolase position. Carbons belonging to the three individual ADP-ribose units are coloured distinctly. (b) Stereoview of an overlay of the modelled endo-glycohydrolase PAR3(colour coded as in panel a) with the observed exo-glycohydrolase crystal structure. Residues implicated in steric hindrance with the additional N+1 unit are shown in VDW spheres (Phe398 and Leu226). The hydrogen network between the N adenosine and the protein/structural water observed for the exo-glycohydrolase binding mode is shown in dotted lines. Figure 3: Model of the PARG–PAR complex in endo-glycohydrolase mode. ( a ) Solvent-accessible surface of PARG in grey (the position of Phe398 is shown in blue) with a PAR 3 modelled in an endo-glycohydrolase position. Carbons belonging to the three individual ADP-ribose units are coloured distinctly. ( b ) Stereoview of an overlay of the modelled endo-glycohydrolase PAR 3 (colour coded as in panel a) with the observed exo-glycohydrolase crystal structure. Residues implicated in steric hindrance with the additional N+1 unit are shown in VDW spheres (Phe398 and Leu226). The hydrogen network between the N adenosine and the protein/structural water observed for the exo-glycohydrolase binding mode is shown in dotted lines. Full size image Table 1 Observed variation of key distances across the MD simulations for a PARG–PAR3 model. Full size table PARG acts mainly as an exo -glycohydrolase The above observations suggest that correct positioning of the n adenosine moiety is indeed important for PARG (exo)glycohydrolase functionality. The mutation of Glu228 to Ala or Ile227 to Pro indeed significantly affects, but does not abolish, TTPARG activity ( Fig. 2a ). This is to be expected for mutations that affect binding affinity but not catalysis, but could also reflect that a proportion of endo-glycohydrolase activity does occur. To further estimate the extent of PARG endo-glycohydrolase activity, we used a mutant bacterial PARG to inhibit the activities of canonical PARG proteins. Unlike eukaryotic PARGs, bacterial PARG shields the terminal n ribose’ from solvent access and was shown to exclusively operate as an exo-glycohydrolase [9] . The Glu115Gln bacterial PARG mutant (corresponding to the Glu256Gln in TTPARG) binds to the PARG reaction product ADP-ribose as efficiently as the wild-type (WT) protein, and it was added in increasing ratios with an aim to protect the substrate PAR termini, gradually allowing for (any residual) endo-glycohydrolase activity only to occur. However, complete inhibition of canonical PARG was observed at higher Glu115Gln concentrations, suggesting that all available PAR termini are protected from PARG exo-glycohydrolase activity ( Fig. 2b ). This suggests that canonical PARG endo-glycohydrolase activity is not comparable to exo-glycohydrolase activity under the conditions used. Detection of PARG endo-glycohydrolase activity has been historically challenging. To overcome this, we developed a sensitive liquid chromatography/mass spectrometry (LC/MS) method that allowed us to detect very low levels of endo-glycohydrolase products. We produced long PAR chains to further increase a chance for endo-glycohydrolitic action. In the conditions used, the PARG reaction enriched the shorter endo products (probably owing to the coupling with exo reaction) and ADP-ribose oligomers of more than four repeats could not be detected ( Fig. 2c ). Bacterial Glu115Gln PARG is also able to inhibit human PARG activity, and our LC/MS data reveal a similar predisposition of the human PARG to generating the ADP-ribose exo-glycohydrolase product, suggesting that canonical PARG activity substrate preferences are conserved across the eukaryotic kingdoms. We generated a Phe398Gly mutation in TTPARG and the corresponding Phe902Gly mutation in human PARG to remove the steric clash that occurs with the poly(ADP-ribose) bound in the endo-glycohydrolase mode. In comparison with the WT human and TTPARG proteins, LC-MS analysis reveals an approximate four- and sevenfold increase of endo-glycohydrolase products, respectively ( Fig. 2c ), supporting the role of Phe398/Phe902 in balancing the relative endo/exo-activities of canonical PARGs. A role for both conserved glutamates in catalysis A model of the TTPARG–PAR Michaelis complex can be derived by positioning the Glu256 in a conformation as observed in the WT TTPARG–ADP-ribose complex (PDB ID:4EPP). This reveals that Glu256 is within the hydrogen bonding distance of the O-glycosidic ribose–ribose bond, thus suggesting that Glu256 is protonated. We performed pK a calculations for the free enzyme and the substrate–TTPARG bound complex. Both Glu255 and Glu256 are predicted to be negatively charged in the free enzyme. Although the predicted pK a of Glu256 does not change substantially for the Glu255Ala mutant in the free enzyme, the charge coupling between both glutamic acid residues is much increased when the substrate is bound such that one proton is added to the pair. As is common for tightly coupled protonations, the precise location of the proton is more difficult to predict, but hydrogen bonding within the active site is consistent with the side chain of Glu256 picking up a proton in the enzyme–substrate complex. Calculations suggest that in the Glu255Ala mutant, where the charge coupling is removed, the Glu256 pK a reverts to a much lower value, and is less likely to pick up a proton. This implies that Glu256 becomes protonated by W2 on PAR binding, and establishes a clear role for Glu255 in the catalytic mechanism that extends beyond the binding of the n ribose’ 2-OH group ( Fig. 4 ). The elevated pK a of Glu256 allows it to protonate the leaving group on concomitant formation of the oxocarbenium intermediate. The Glu256-mediated hydrolysis of this intermediate can then occur either by W1 (which is within the hydrogen bonding distance of the ribose’ C2) or by W2. Modelling studies indicate that the motion of W1 is severely restricted compared with W2, and thus it seems plausible that the latter is responsible for PAR hydrolysis, leading to the α-ribose product. 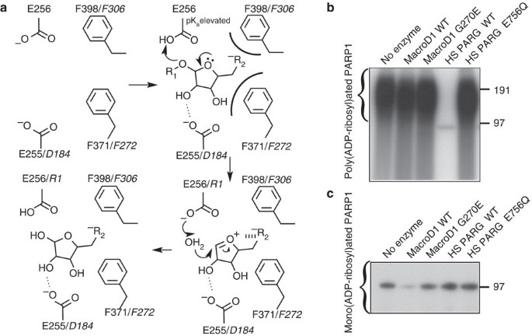Figure 4: A mechanism for poly-ADP-ribose hydrolysis. (a) A detailed mechanism for PARG and MacroD1 based on the PARG-PARG structure. R1=pADPr for PARG, glutamate for MacroD1 and R2=ADP. (b) PARG is unable to hydrolyse the terminal ADP-ribose–PARP1 bond. MacroD1 and human PARG activities on radioactively labelled poly(ADP-ribosyl)ated PARP1. MacroD1 WT and the catalytic mutant, G270E, as well as human PARG E756Q mutant, are unable to process PAR. (c) MacroD1 WT removes the terminal ADP-ribose group attached to mono(ADP-ribosyl)ated PARP1 E988Q substrate. In contrast, the MacroD1 catalytic mutant and human PARG do not exhibit the mono(ADP-ribosyl) hydrolase activity. Figure 4: A mechanism for poly-ADP-ribose hydrolysis. ( a ) A detailed mechanism for PARG and MacroD1 based on the PARG-PARG structure. R1=pADPr for PARG, glutamate for MacroD1 and R2=ADP. ( b ) PARG is unable to hydrolyse the terminal ADP-ribose–PARP1 bond. MacroD1 and human PARG activities on radioactively labelled poly(ADP-ribosyl)ated PARP1. MacroD1 WT and the catalytic mutant, G270E, as well as human PARG E756Q mutant, are unable to process PAR. ( c ) MacroD1 WT removes the terminal ADP-ribose group attached to mono(ADP-ribosyl)ated PARP1 E988Q substrate. In contrast, the MacroD1 catalytic mutant and human PARG do not exhibit the mono(ADP-ribosyl) hydrolase activity. Full size image PARG does not hydrolyse mono-ADP-ribosylated substrates Modelling of a glutamate linkage to the n ribose’, to mimic the protein-PAR linkage, leads to clashes of the glutamate carboxylate moiety with PARG Val253 and Ala370. Furthermore, the presence of non-catalytic domains of PARG (the accessory domain and the additional regulatory domain in mammalian PARGs) probably limits access to the active site for bulkier ADP-ribosylated protein substrates. It has recently been established that several macrodomain proteins namely MacroD1, MacroD2 and TARG1 (refs 16 , 17 , 18 ) can catalyse the removal of the final ADP-ribose moiety efficiently ( Fig. 4b ). A comparison of the MacroD1 and MacroD2 structures [17] , [21] with the PAR-PARG complex ( Supplementary Fig. S5 ) reveals that it does not contain the PARG-specific catalytic loop insert and associated additional domains, rendering the MacroD1/D2 active site significantly more accessible to the ADP-ribosylated protein. Furthermore, unlike for the hydrolysis of the O-glycosidic ribose–ribose linkage, the formation of the oxocarbenium intermediate in hydrolysis of the glutamate–ADP-ribose linkage does not require acid–base catalysis. We propose that MacroD1 and related proteins catalyse bond breakage by forcing the substrate ribose’ close to the α-phosphate, similar to what has been suggested for PARG. Although the MacroD1/D2 and PARG structures share similarities in the binding mode of the ADP-ribose module, the related non-catalytic MacroH2A.1.1 (ref. 22 ) has a distinct conformation for the ribose’, supporting the notion that enzymatic macrodomains achieve catalysis by inducing substrate strain. It has been suggested that in MacroD1/D2 a conserved structural water molecule, positioned between the ribose and the alpha-phosphate, could be activated by the latter. In view of the established pK a of α-phosphates of~2 (ref. 21 ), this seems unlikely. In the absence of any obvious MacroD1/MacroD2-derived acid–base catalyst, it is possible that the Glu leaving group is involved in assisting hydrolysis of the oxocarbenium intermediate or that non-enzymatic hydrolysis of the unstable intermediate occurs. The TTPARG–PAR 9 complex crystal structure represents the first visualization of PAR binding at atomic detail and encourages further structural studies aimed at understanding PAR-protein interaction networks involved in genome stability. Supported by biochemical and modelling studies, the structural data indicate that canonical PARG is inherently predisposed to act as an exo -glycohydrolase owing to higher affinity for the PAR terminus, a consequence of the presence of the conserved phenylalanine residue (Phe398/902). Unlike the bacterial PARG, however, a (latent) low-affinity endo- glycohydrolase binding mode is possible, as confirmed by our LC-MS studies of the WT proteins. This suggests that, in vivo , the relative balance between exo- and endo- glycohydrolase activity will be a function of the PAR/PARG ratio. The latter mode of action is more likely in cases where PAR/PARG ratio is increased, for instance, when cells encounter extreme stress leading to excess PAR production and apoptosis, where released larger oligo-PAR fragments may act to further amplify the apoptotic signal [23] . We suggest that under normal physiological conditions ADP-ribose is the dominant PARG product, with the latent endo-glycohydrolase activity of PARG activated by increased PAR/PARG ratios and/or increasing PAR chain lengths following cellular insult. The final step in complete removal of PAR requires hydrolysis of the glutamate–ADP-ribose linkage connecting PAR to the modified protein. This reaction is catalysed by MacroD family of proteins (in addition to TARG1), which do not contain the PARG-specific acid–base catalytic machinery, but make similar use of substrate strain to catalyse the formation of the oxocarbenium intermediate. Plasmids and proteins The WT and mutant T. thermophila PARG2 (TTHERM_00294690) were expressed from the pET28a vector (Novagen). Human PARG with an N-terminal truncation (Δ1–455) served as a reference for the WT PARG activity, and the mutant PARG constructs were expressed from the pColdTF vector (Takara). All proteins bear an N-terminal his-tag. For crystallization studies, T. thermophila E256Q mutant was purified by fast protein liquid chromatography (FPLC) on a HisTrap HP column (GE Healthcare), followed by size-exclusion chromatography using HiLoad 16/60 Superdex 200 column. Mutations were introduced using the QuickChange II Site-Directed Mutagenesis kit (Stratagene). PARG activity assays For western blot analysis of PARG activity, PAR was synthesized by the automodification of PARP1 in a reaction mixture containing 2 units of PARP1 (Trevigen), 200 μM NAD (Trevigen), activated DNA (Trevigen), 50 mM Tris (pH 7.5) and 50 mM NaCl at room temperature. Reactions were stopped after 30 min by the addition of the PARP inhibitor KU-0058948 and contain 5 μM of PAR. In mutational studies, either 80 nM human NTR1 or 7 nM T. thermophila WT and mutant PARGs were added to the reactions and incubated for another 30 min. In PARG inhibition studies, a preincubation step with T. curvata E115Q (ref. 9 ) was included. In the latter assays, the reaction mix was incubated with increasing amounts (0.05, 0.1, 0.5, 0.75, 1, 2, 5 and 10 μM) of T.curvata E115Q PARG for 5 min before the addition of 20 nM human full-length or 30 nM T. thermophila PARGs, followed by a subsequent 15-min incubation at room temperature. All reactions were run on 4–12% SDS–PAGE gels and blotted onto a nitrocellulose membrane. PAR hydrolysis was visualized by rabbit polyclonal anti-PAR antibodies (Trevigen; 1:1,000 dilution). Western blots were analysed densitometrically by GeneTools (SynGene), followed by statistical analysis using a paired t -test. PAR isolation and analytical verification PAR biosynthesized by tankyrase 1 (1,093–1,327) in the presence of histones were detached with potassium hydroxide and purified by means of the dihydroxy boronyl column. The resulting bulk polymers were fractionated by anion exchange chromatography and desalted to yield PAR of defined lengths [20] . Crystallization and structure solution A concentration of 15.5 mg ml −1 TTPARG E256Q was incubated with a series of purified PAR fragments at 1 mM (hexamer, heptamer, decamer, tetradecamer and pentadecamer were used) before setting down sitting-drop vapour diffusion trays. Crystals were observed for all PAR fragments tested under a range of conditions. Crystals were flash-cooled in liquid nitrogen, and diffraction data were collected at the Diamond Lightsource (UK), reduced and scaled using X-ray Detector Software (XDS) [24] . The highest resolution data were obtained for a PAR9 complex, which was obtained in 0.1 M HEPES, pH 7.0, and 30% v/v Jeffamine ED-2001 at 4 °C. The structure was solved by molecular replacement using the WT TTPARG structure [10] (PDB ID: 4EPP), and final refinement statistics are given in Table 2 . Table 2 Crystallographic data and model refinement parameters. Full size table Molecular dynamics simulations Topology and parameter files for the PAR trimer were obtained using the Antechamber program [25] with AM1-BCC charges [26] . The PARG–ligand complex model was placed in a periodic water box (TIP3) and neutralized by adding Na + ions. This complex was equilibrated with several cycles of minimizations (steepest descent, 10,000 steps) and MD simulations (50 K, 20 ps) with the protein atoms fixed. MD simulations were performed (310 K, 0.5 ns) at a time step of 2 ps, with the protein backbone restrained to the X-ray structure conformation. Individual snapshots showing the PARG–ligand interactions were extracted from the last 100-ps simulation, and minimized (10,000 steps, steepest descent). The overall r.m.s.d. of the PAR endo –PARG model with the X-ray coordinates was 0.43 Å for all Cα atoms. pK a calculations Calculations of pK a values were made with a combined Finite Difference Poisson–Boltzmann and Debye–Hückel method, termed FDDH [27] , [28] . Relative dielectric values of 78.4 (water) and 4 (protein, Finite Difference Poisson–Boltzmann method) were assigned, with an ionic strength of 0.15 M. Calculations were made for TTPARG with and without the bound PAR substrate. Ultrahigh-performance liquid chromatography coupled to quadrupole time-of-flight mass spectrometry The poly(ADP-ribosyl)ated PARP1 was treated with PARG, and the mixture was filtered using centricons (30 kDa cutoff). The analysis of the filtrate was performed using a modified procedure by Coulier et al. [29] , as described earlier in Dunstan et al . [10] Briefly, all analyses were performed using a Waters Acquity ultrahigh-performance liquid chromatography system (Waters, Milford, MA, USA), equipped with a binary solvent delivery system and autosampler. The chromatographic separations used a column (100 mm × 2.1 mm) filled with a 1.7 μm BEH C 18 stationary phase (Waters, Milford, MA, USA). Binary gradients at a flow rate of 0.4 ml min −1 were applied for the elution. The eluent A was water containing 5 mmol l −1 of pentylamine, and the pH value was adjusted to 6.5 using acetic acid, whereas the eluent B was acetonitrile. A fast elution gradient was applied, starting with 2% B, and then the percentage of B linearly increased to 25% in 5 min, followed by an isocratic hold until 10 min. The mass spectrometry was performed on a quadrupole time-of-flight Premier instrument (Waters Micromass, Manchester, UK) using an orthogonal Z-spray–electrospray interface. The instrument was operated in V mode, with time-of-flight mass spectrometry data being collected between m/z 100 and 2,000, applying collision energy of 4 eV. All acquisitions were carried out using an independent reference spray via the lock spray interface, whereas leucine enkephalin was applied as a lock mass in negative ionization mode ( m/z 554.2615). The reaction products, expected to occur in the reaction mixture, in particular ADP-ribose and oligomers of poly-ADP-ribose with up to five ADP-ribose units, as well as NAD + , were searched for using extracted ion chromatograms. The target analyses were based on the characteristic accurate m/z ratios applying a mass window of 50 mDa. As the information on the electrospray ionization mass spectra for oligomeric ADP-ribose species are only scarcely available in the literature [30] , the recorded total ion current (TIC) chromatograms were systematically examined using specific masses of possible mono- and multiply charged ions of individual oligomers. The optimal responses were obtained using m/z ratios of 558.0639, 1,099.125, 819.589 and 1,090.120 for deprotonated ADP-ribose, deprotonated ADPR dimer, doubly charged deprotonated ADPR trimer and doubly charged deprotonated ADPR tetramer, respectively. The relative contributions of the individual oligomers were determined assuming that they had the same responses as ADPR. Accession codes : Coordinates and structure factors for catalytically inactive PARG in complex with a poly(ADP-ribose) fragment have been deposited in the protein data bank under PDB accession code 4L2H . How to cite this article: Barkauskaite, E. et al. Visualization of poly(ADP-ribose) bound to PARG reveals inherent balance between exo- and endo-glycohydrolase activities. Nat. Commun. 4:2164 doi: 10.1038/3164 (2013).